Structural origins of Johari-Goldstein relaxation in a metallic glass Johari-Goldstein or β relaxation, persisting down to glassy state from a supercooled liquid, is a universal phenomenon of glassy dynamics. Nevertheless, the underlying micromechanisms leading to the relaxation are still in debate despite great efforts devoted to this problem for decades. Here we report experimental evidence on the structural origins of Johari-Goldstein relaxation in an ultra-quenched metallic glass. The measured activation energy of the relaxation (~26 times of the product of gas constant and glass transition temperature) is consistent with the dynamic characteristics of Johari-Goldstein relaxation. Synchrotron X-ray investigations demonstrate that the relaxation originates from short-range collective rearrangements of large solvent atoms, which can be realized by local cooperative bonding switch. Our observations provide experimental insights into the atomic mechanisms of Johari-Goldstein relaxation and will be helpful in understanding the low-temperature dynamics and properties of metallic glasses. Johari-Goldstein (JG) relaxation has intrinsic correlation with glass transition and many fundamental properties of glassy materials [1] , [2] , [3] , [4] , [5] . It is generally explained in term of hindered intra- and/or inter-molecular motion that remains active even when the whole system is frozen into the glassy state [1] . However, the underlying micromechanisms leading to JG relaxation have not been fully understood [2] , [3] , [4] , [5] , [6] , [7] , [8] , [9] , [10] , [11] , [12] , [13] , mainly because of the lack of well-defined experimental characterization on the structural evolution of the disordered glasses. It remains indistinct that the relaxation is essentially involved all atoms/molecules that happens spatially uniformly or originates from local atomic rearrangement associated with structural and chemical heterogeneity [2] , [3] , [11] , [12] , [13] , [14] , [15] , [16] . Different from organic and net-work oxide glasses, metallic glasses are basically atomic glasses with fundamental components of individual atoms and can be treated as randomly packed hard spheres without complex inter- and intra-molecular interactions. Besides their technical importance for a wide range of applications, metallic glasses are also an ideal system for understanding the basic physical process of structural relaxation in glassy solids on an atomic scale. Since the relaxation of conductive metallic glasses cannot be studied using dielectric spectroscopy, JG relaxation in metallic glasses is mainly characterized by differential scanning calorimetry (DSC) [7] , [8] , [16] and dynamical mechanical spectroscopy [9] , [10] , [17] , [18] . Unlike spectroscopic method, the DSC measurements are an out-of-equilibrium and nonlinear approach. JG relaxation is superimposed on the broad sub- T g exothermic relaxation patterns that are the direct outcome of combined secondary and primary relaxations, while JG relaxation appears at the low-temperature side as the tails of the primary relaxation bands [7] , [8] , [16] . It has been suggested that the relaxation of metallic glasses depends on fragility, cooling rate, chemical bonding, atomic size disparity and constitute atom diffusivity [3] , [8] , [9] , [16] , [17] , [18] , [19] . Since these kinetic and chemical variables are essentially associated with structure of metallic glasses, directly investigating the correlation between atomic structure and JG relaxation may shed a light on the atomic origins of the low-temperature relaxation. However, metallic glasses usually have a weak JG relaxation in proportion to trivial structure evolution because the high atomic mobility gives rise to fast structure relaxation during cooling from liquid to glass state. Although it has been noticed that the intensity of JG relaxation can be enhanced by high cooling rates [16] , [20] , the intensity enhancement from the currently feasible rapid quenching techniques, such as melting spinning, is still insufficient for detectable structure changes because of the maximum cooling rate is only ~10 6 K s −1 . In this study we developed an ultra-quenched metallic glass with an ultrahigh cooling rate of ~3.6 × 10 9 K s −1 which is ~3–6 orders of magnitude higher than conventional metallic glasses. The ultrahigh cooling rate effectively freezes the glass at a high-energy state with a high fictive temperature and, hence, amplifies JG relaxation for structure study. The measured activation energy for the low-temperature relaxation of the ultra-quenched metallic glass, ~1.39 eV (~26 RT g , where R is the gas constant and T g is the glass transition temperature), is consistent with the characteristics of JG relaxation. Systematic structural characterization using synchrotron X-ray scattering demonstrates that the JG relaxation mainly arises from short-range configuration transformation of solvent atoms by local cooperative bonding switch. 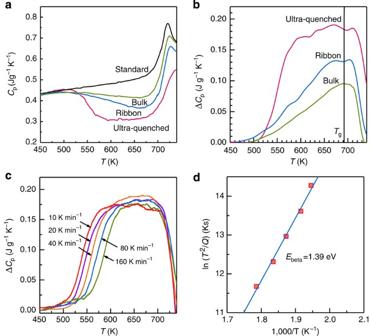Figure 1: Thermal characterizations with differential scanning calorimetry. (a) Apparent heat capacityCp of the ultra-quenched, ribbon, bulk and standard samples. (b) Activation spectra of the three glass samples that experienced high cooling rates. (c) Activation spectra of the ultra-quenched glass measured at different heating rates. (d) Kissinger plot of the onset temperature versus heating rate for the secondary relaxation. Thermal measurements Figure 1a presents the apparent heat capacity, C p , during the first up-scan of the ultra-quenched film, ribbon and bulk glass samples, as well as that of the second up-scan of the slowly cooled specimen within DSC at the rate of 0.33 K s −1 (defined as the standard sample as the reference). The DSC curves indicate that there is a weak cooling rate dependence of the DSC glass transition temperatures ( T g ) of the four samples upon heating. The mean value of T g is ~690 K. Different from the standard sample, broad exothermic peaks can be seen from the film, ribbon and bulk glass samples that experienced faster cooling. The release of the trapped enthalpy by the JG relaxation starts at an onset temperature of ~500 K, which is independent of cooling rates. However, the amplitudes of the JG relaxation show the strong dependence on the cooling history of the samples. Compared with the ribbon and bulk samples, the film exhibits a much more pronounced ΔC p peak ( Fig. 1b ), where ΔC p characterizes the heat capacity difference between the as-prepared and the standard samples. As illustrated in Fig. 1c , the relaxation peak of the film shifts to higher temperatures with heating rates increasing, indicating the strong rate dependence of the JG relaxation. Figure 1d is the Kissinger plot of the onset temperatures ( T c ) of the relaxation at different heating rates. The measured activation energy, E beta , is determined to be 1.39 eV, which is well consistent with the reported values of Zr-based glasses obtained by the enthalpy relaxation approach [8] . It is worth noting that the E beta value is in accordance to the universal activation energy (~26 RT g ) of JG relaxation, the dynamic characteristics widely observed in glassy materials [8] , [9] , [16] , [17] , [18] , [21] , [22] . Although the broad sub- T g exothermic peak in the DSC traces of the ultra-quenched metallic glasses may be the outcome of combined JG and primary relaxations together with other possible sources, such as irreversible structural relaxation, the dynamic identity of the activation energy provides the solid evidence that the low-temperature side of relaxation spectra and the onset of C p mainly originate from JG relaxation, while the contribution of the structural relaxation is minor. Figure 1: Thermal characterizations with differential scanning calorimetry. ( a ) Apparent heat capacity C p of the ultra-quenched, ribbon, bulk and standard samples. ( b ) Activation spectra of the three glass samples that experienced high cooling rates. ( c ) Activation spectra of the ultra-quenched glass measured at different heating rates. ( d ) Kissinger plot of the onset temperature versus heating rate for the secondary relaxation. Full size image We evaluated the energy states of the glassy samples by calculating their fictive temperatures, T f , at which the structure of the equilibrium liquid is frozen into a glass state. According to the energy matching method [23] , T f can be derived by equalling the area hatched by the heat capacity curves of the first ( C p1 ) and second ( C p2 ) up-scans to that enclosed by C pl and C pg from T g to T f —that is, , where T c is the temperature at which energy release starts; T eq is the temperature where the equilibrium liquid is reached; C pl and C pg are the heat capacities of the supercooled liquid and glass, respectively. On the basis of the equation, the fictive temperatures of the ribbon and bulk glasses are calculated to be 1.21 T g and 1.11 T g , respectively, in line with the typical values of conventional metallic glasses. For the ultra-quenched film glass, the T f is as large as 1.34 T g , approaching the melting temperature T m of the alloy ( T f =0.83 T m ), verifying that the film glass is trapped at a high-energy state far away from equilibrium. 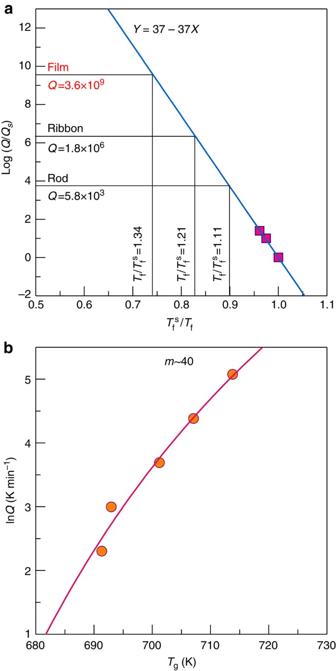Figure 2: Determination of fictive temperatures. (a) Scaled Arrhenius plot of fictive temperature and cooling rate. (b) Dependence of glass transition temperature on heating rate. The solid line is the Vogel–Fulcher–Tamman equation fitting to the data points. Figure 2a shows the Arrhenius plot of the scaled cooling rate Q/Q s and fictive temperature T f / by the standard sample. Since the standard sample experienced a constant slow rate of Q s =0.33 K s −1 on cooling and heating, its fictive temperature is approximately equal to T g (=690 K). The nominal cooling rates of the glasses can be determined by the scaled Arrhenius plot on the basis of their estimated fictive temperatures in a calibration line [24] . In addition to the standard sample with the cooling rate of 0.33 K s −1 and fictive temperature of 690 K, the calibration line is constructed by the designed cooling rates of 8.33 and 3.33 K s −1 using DSC. According to the derived T f values, the cooling rate of the film is as high as ~3.6 × 10 9 K s −1 , about 3 and 6 orders of magnitude higher than that of the ribbon (1.8 × 10 6 K s −1 ) and bulk (5.8 × 10 3 K s −1 ) samples. The slope of the plot in Fig. 2a yields the fragility ( m ) of ~37, which is related to the activation energy E a for glass transition by m = E a /2.303 RT g (ref. 24 ). The fragility ( m =37) is in the good agreement with that ( m =40) obtained by measuring the heating rate dependence of T g ( Fig. 2b ) [25] , validating that the T f and cooling rates determined from the calibration line are dependable. Figure 2: Determination of fictive temperatures. ( a ) Scaled Arrhenius plot of fictive temperature and cooling rate. ( b ) Dependence of glass transition temperature on heating rate. The solid line is the Vogel–Fulcher–Tamman equation fitting to the data points. Full size image Synchrotron X-ray diffraction characterization We utilized synchrotron radiation X-ray diffraction (XRD) and the extended X-ray absorption fine structure (EXAFS) spectroscopy to experimentally investigate the structural evolution of the glassy samples caused by JG relaxation. 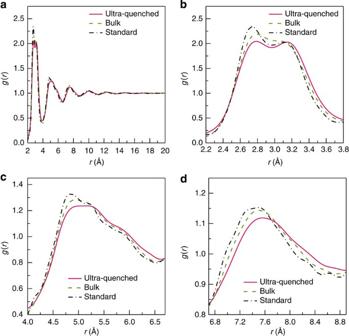Figure 3: Pair distribution functions derived from synchrotron XRD. (a) The overall tendency of the pair distribution functions. (b–d) Close inspections of the first, second and third peaks of PDFs. Figure 3a displays the pair distribution functions (PDFs), g ( r ), of ultra-quenched, bulk and standard glasses, which were derived from XRD data. The PDFs reveal short to medium-range ordering up to ~15 Å, beyond which conspicuous correlation peaks cannot be observed. Close inspection indicates that the first peaks of the Zr 55 Cu 30 Ni 5 Al 10 glasses split into two sub-peaks locating at ~2.80 and 3.15 Å ( Fig. 3b ) due to the discrete bonding length distribution of the nearest neighbour atoms. According to the Goldschmidt radii and weight factors ( Table 1 ), the first sub-peak can be assigned mainly to the Zr-Cu pairs, while the Zr-Zr pairs dominate the second sub-peak. The large weight factor of the Zr-Cu pairs is consistent with the fact that the Cu-centred clusters are the dominant short-range order as demonstrated by molecular dynamics simulation [26] . Compared with the standard and bulk samples, the ultra-quenched film shows obviously higher g ( r ) Zr-Zr / g ( r ) Zr-Cu ratio, indicating more Zr-Zr pairs and lesser Zr-Cu pairs in the sample. By integrating the first peak of the PDFs, the average coordination numbers are found to be ~13.6 for all the three glasses, indicating very small variation in the global average coordination numbers. The cooling rate-induced difference in the coordination number is probably too small to be identified. However, the expanded width of the first peak of the film suggests that the atomic packing in the nearest neighbours is looser compared with the standard and bulk samples ( Fig. 3b ), which coincides with the high fraction of the longer Zr-Zr pairs. For the second and third peaks of the film glass, substantial peak broadening cannot be seen. Instead, their intensities are noticeably lower than those of the standard sample ( Fig. 3c,d ). This indicates the loss of medium-range order in the ultra-quenched film glass, which is presumably due to the expanded nearest neighbours that cause the structure frustration beyond the first shells [27] . Figure 3: Pair distribution functions derived from synchrotron XRD. ( a ) The overall tendency of the pair distribution functions. ( b – d ) Close inspections of the first, second and third peaks of PDFs. Full size image Table 1 Inter-atomic bond lengths and weight factors of atomic pairs in the Zr 55 Cu 30 Ni 5 Al 10 metallic glass. Full size table EXAFS results The local atomic structure of the glass samples is further characterized by EXAFS, which is highly sensitive to local elemental specificity. 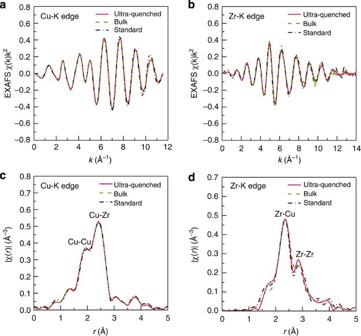Figure 4: EXAFS spectra of the ultra-quenched, bulk and standard samples. (a)k2χ(k) spectra of Cu-K-edge; and (b) Zr-K-edge. (c) Fourier transform profiles of the experimental EXAFS spectra of Cu-K-edge, and (d) Zr-K-edge. Figure 4a,b shows the EXAFS k 2 χ( k ) spectra of Cu-K and Zr-K edges from ultra-quenched, bulk and standard glass samples, respectively. The spectra of the three samples at the Cu-K edge are nearly identical, indicating that the huge cooling rate difference among the samples does not cause detectable changes in the nearest neighbours of Cu atoms. However, at the Zr-K edge the spectrum of the ultra-quenched glass shows detectable difference from the bulk and standard samples, particularly at the low- k region. The Fourier transform profiles of k 2 χ( k ) spectra of Cu and Zr-K edges are shown in Fig. 4c,d . Two sub-peaks, corresponding to Cu-Cu and Cu-Zr pairs, can be seen in the Cu-K-edge spectra ( Fig. 4a ), signifying that the first shell of the Cu-centred clusters includes both Cu and Zr solvent atoms. While the standard specimen is almost fully relaxed in comparison with the ultra-quenched glass, its peak intensity ratio between Cu-Cu and Cu-Zr pairs remains the nearly same as those of the samples with higher cooling rates. This indicates that the pronounced JG relaxation of the film glass does not entail visible alteration of the local chemical environments of the prevalent Cu-centred polyhedra in the metallic glass. In contrast, the Fourier transform of the Zr-K edge k 2 χ( k ) spectra shows the noticeable difference of the ultra-quenched glass from the bulk and standard ones in the magnitude ratios of the peaks of Zr-Zr and Zr-Cu pairs ( Fig. 4d ). As the peak magnitude ratio corresponds to the number fraction of neighbouring atoms, considering the inconspicuous difference in the Fourier-transformed Cu-K edges of the three samples ( Fig. 4c ), it can be concluded that the fraction of Zr-Cu pairs (2.85 Å) evidently increases, while that of longer Zr-Zr pairs (3.16 Å) decreases in the relaxed standard and bulk sample. This local chemical measurements are fully consistent with the statistic geometry analysis by XRD ( Fig. 3b ) in which the Zr-Zr pairs have a higher fraction than that of Zr-Cu in the ultra-quenched film. Figure 4: EXAFS spectra of the ultra-quenched, bulk and standard samples. ( a ) k 2 χ( k ) spectra of Cu-K-edge; and ( b ) Zr-K-edge. ( c ) Fourier transform profiles of the experimental EXAFS spectra of Cu-K-edge, and ( d ) Zr-K-edge. Full size image To further verify the local structural changes mainly originating from JG relaxation, we investigate the atomic configuration evolution of the isothermally annealed ultra-quenched glass at 623 K, close to the peak temperature of JG relaxation, for 30 min and 12 h. Since this temperature is far below T g (690 K), the primary relaxation (glass transition) and irreversible structural relaxation should not take place. The EXAFS k 2 χ( k ) spectra of Cu-K and Zr-K edges from the annealed ultra-quenched glass films are presented in Fig. 5a,b , while their Fourier transform profiles are displayed in Fig. 5c,d . As seen from the Cu-K edge, the peak positions as well as the magnitude ratios of the Cu-Cu and Cu-Zr pairs remain constant with the annealing time increasing from 30 min to 12 h ( Fig. 5c ). Nonetheless, the isothermal annealing-induced structure changes are visible from the Zr-K edge. The intensity magnitude of the Zr-Zr peak detectably decreases with annealing time ( Fig. 5d ), further confirming that JG relaxation mainly involves the reduction of solvent Zr-Zr pairs. 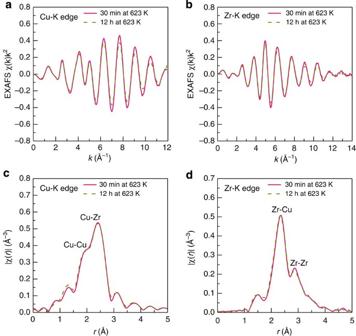Figure 5: EXAFS spectra of the ultra-quenched glass annealed at 623 K. (a)k2χ(k) spectra of Cu-K-edge; and (b) Zr-K-edge. (c) Fourier transform profiles of the experimental EXAFS spectra of Cu-K-edge, and (d) Zr-K-edge. Figure 5: EXAFS spectra of the ultra-quenched glass annealed at 623 K. ( a ) k 2 χ( k ) spectra of Cu-K-edge; and ( b ) Zr-K-edge. ( c ) Fourier transform profiles of the experimental EXAFS spectra of Cu-K-edge, and ( d ) Zr-K-edge. Full size image Both XRD and EXAFS characterizations demonstrate that very local chemical ordering around the solvent Zr atoms takes place during JG relaxation. The reduced number fraction of Zr-Zr pairs during the JG relaxation is expected to lead to the formation of more Cu-centred polyhedra. Although we cannot detect the Al- and Ni-related atomic pairs because of their low weight factors ( Table 1 ), the EXAFS analysis demonstrates that the local structure changes during JG relaxation mainly arise from the local rearrangement of the solvent Zr atoms with a larger size, whereas the chemical constitution of the dominant Cu-centred clusters remain nearly unaffected. On the basis of the XRD and EXAFS measurements, the key structure changes of the film glass upon JG relaxation can be summarized as the following: (1) the packing density of the nearest neighbours increases as evidenced by the difference in the first peak widths of the PDF profiles ( Fig. 3b ); and (2) the number fraction of Zr-Zr atomic pairs in the nearest neighbours of Zr atoms decreases by substitution of Zr-Cu pairs, while the prevailing Cu-centred clusters do not show too much change in the number of solvent Zr atoms. Therefore, the physical process of JG relaxation of the ultra-quenched glass is apparently associated with a local atomic rearrangement beyond the dominant Cu-centred clusters and only solvent atoms, mostly Zr atoms, are rearranged by a short-range collective process. There are many possible dynamic paths to realize the local structure changes during JG relaxation. The most feasible one is probably by a simple bonding switch as depicted in Fig. 6 . This easy cooperative atomic rearrangement can give rise to the key structure changes revealed by XRD and EXAFS—that is, the decreased Zr-Zr inter-atomic pairs (correspondingly, increased Zr-Cu pairs) and denser atomic packing. Since Zr atoms have a large atomic size and typically locate at the shells of densely packing clusters or adjunct sites between these clusters, some of them may be dynamically too slow to travel to a low-energy basin during fast quenching and hence are trapped in a high-energy state by bonding with other Zr atoms ( a of Fig. 6 ). The JG relaxation process can be accomplished by a simple bonding switch from a long Zr-Zr pair to a tight Zr-Cu one through a cooperative short-range atomic motion as shown in b of Fig. 6 . This process leads to the formation of a densely packed Cu-centred cluster and the loss of a long Zr-Zr pair. It is analogous to shear-induced bonding switch [28] but, however, the difference is also obvious since the bonding switch during JG relaxation is solely assisted by thermal fluctuation at high temperatures and can be revisable by being quenched from the same fictive temperature of the glass. The short-range collective rearrangement of solvent atoms leads to the increased packing density, while the chemical environments of individual Cu-centred clusters are not affected except the increase in their number density, which will not lead to any changes in the EXAFS Cu-K edge profiles. 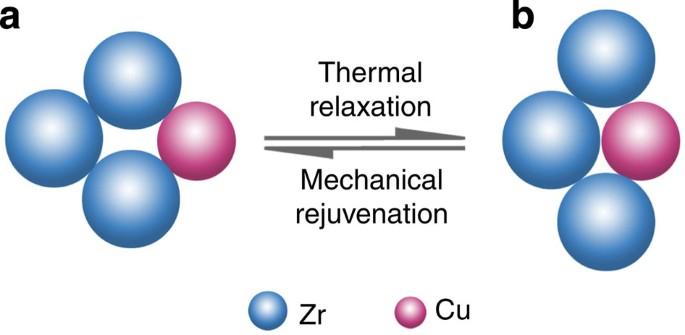Figure 6: Schematic diagram of secondary relaxation by local bonding switch. The break of the long Zr-Zr pair distance and formation of the short Zr-Cu bond lead to the denser local atomic packing. Figure 6: Schematic diagram of secondary relaxation by local bonding switch. The break of the long Zr-Zr pair distance and formation of the short Zr-Cu bond lead to the denser local atomic packing. Full size image As illustrated by this study, JG relaxation mainly originates from the local structure transformation associated with large solvent atoms. This appears to be in contradiction of the recent report on the coupling of small atoms diffusion with JG relaxation in metallic glasses [9] . In fact, the two observations tell the same scenario but from different aspects that are emphasized. Our structure characterization reveals the atomic configuration changes upon JG relaxation, while the activation energy measurement by Yu et al . [9] discloses the dynamic process of high mobility of small atom resulted from JG relaxation. As shown in the bonding switch model ( Fig. 6 ), the resultant structure changes, corresponding to JG relaxation, are accomplished by the collective rearrangements of large solvent atoms. However, the dynamic process of the collective atomic transformation is mainly realized by the motion of smaller atoms over a short range—for example, Cu in this study—because of their high mobility and coordination capacity of filling the excess open space among the large solvent atoms. It has been noticed that JG relaxation at a temperature below T g gives rise to significant change in the volume of shear transformation zones (STZs) [10] , the basic flow units in metallic glasses. Although it has been long known that STZs are associated with heterogeneous atomic packing in metallic glasses [29] , the physical process of STZ formation is very vague and lacks distinct physical description. As the barrier energy of STZs is also equal to the activation energy of JG relaxation, it is rational to deduce that STZs share the same physical process with JG relaxation [12] . STZs may initiate from the regions with loosely packed solvent atoms, consistent with previous molecular dynamics simulations [30] , and are dynamically manipulated by stress-induced atom motion. Accordingly, the STZ formation may be considered as the result of dynamic coupling between applied stress and inherent structure relaxation. In summary, we developed an ultra-quenched metallic glass that undergoes a cooling rate on the order of ~10 10 K s −1 . The glass shows pronounced sub- T g relaxation compared with conventional ribbon and bulk glasses. The measured activation energy demonstrates that the relaxation has the dynamic characteristics of JG relaxation. Atomic structural characterization suggests that the relaxation originates from short-range collective rearrangements of solvent atoms beyond densely packed atomic clusters. This study may shed light on the atomic mechanisms of JG relaxation and bear important implications on the structural process of plastic deformation in glassy metals. Sample preparation The ultra-quenched Zr 55 Cu 30 Ni 5 Al 10 metallic glass was fabricated by means of rf-magnetron sputtering deposition [31] . To acquire sufficient DSC and XRD signals, ~30-μm thick glassy films were prepared with the well-controlled sample temperature below 50 °C. Ribbon and bulk glasses with the same chemical composition were made by conventional melt-spinning and copper-mold-casting methods, respectively. Slowly cooled samples were prepared by reheating the glassy sample to the supercooled liquid region and then cooling to ambient temperature at the rate of 20 K min −1 . DSC measurements Thermal analysis was conducted by using a Perkin-Elmer 8500 DSC with which controllable cooling rate can be achieved up to 500 K min −1 . The samples were first heated to their supercooled liquid region at the rate of 20 K min −1 to obtain the heat capacity traces ( C p1 ) of the as-prepared samples, and then slowly cooled at the same rate to room temperature. The slowly cooled samples were then subjected to the second up- and down-scan following the same procedure to establish the standard heat capacity curves ( C p2 ). Structural characterization The structural characterization was performed at SPring-8 synchrotron radiation facility, Japan. High-energy XRD with the beam energy of 113.3 keV was carried out in transmission geometry. The diffraction data were analysed following the procedures in Kohara et al . [32] The local atomic structure of the samples was characterized by the EXAFS spectroscopy [33] . EXAFS measurements of the Cu and Zr-K edges were conducted in a transmission mode at the bending magnet beam line BL01B1 of the synchrotron radiation facility (SPring-8) in Hyogo, Japan. Incident X-ray energy was selected by a fixed-exit double-crystal monochromator using Si(111) planes for the Cu-K-edge and the Zr-K-edge. EXAFS oscillation functions χ( k ) and their magnitude of Fourier transforms χ(r) are deduced from the EXAFS spectra using a coded program of Athena [34] . The energy edge ( E 0 ) was set to a set fraction (50%) of the edge step. The k -range of forward Fourier transform is from 2 to 11 Å −1 for both Cu-edges and Zr-edges. It is common practice in EXAFS to multiply χ( k ) by different k -weights. In this study, we used k 2 to calculate χ(r) (Å −3 ). How to cite this article: Liu, Y. H. et al . Structural origins of Johari-Goldstein relaxation in a metallic glass. Nat. Commun. 5:3238 doi: 10.1038/ncomms4238 (2014).